Measurement of acetylation turnover at distinct lysines in human histones identifies long-lived acetylation sites Histone acetylation has long been determined as a highly dynamic modification associated with open chromatin and transcriptional activation. Here we develop a metabolic labelling scheme using stable isotopes to study the kinetics of acetylation turnover at 19 distinct lysines on histones H3, H4 and H2A. Using human HeLa S3 cells, the analysis reveals 12 sites of histone acetylation with fast turnover and 7 sites stable over a 30 h experiment. The sites showing fast turnover (anticipated from classical radioactive measurements of whole histones) have half-lives between ~1–2 h. To support this finding, we use a broad-spectrum deacetylase inhibitor to verify that only fast turnover sites display 2–10-fold increases in acetylation whereas long-lived sites clearly do not. Most of these stable sites lack extensive functional studies or localization within global chromatin, and their role in non-genetic mechanisms of inheritance is as yet unknown. In eukaryotic cells, 147 bp of DNA is tightly wrapped around a histone octamer, consisting of one copy of H3-H4 tetramer and two copies of H2A-H2B dimer, to form the nucleosome. In the ‘beads on a string’ model, the repeating nucleosomes and flanking ‘linker’ DNA form a 10-nm-fibre with histone H1 stabilizing the structure. It has been suggested that a chain of nucleosomes is further folded into a 30-nm fibre in the so called ‘solenoid’ or ‘double start’ structure [1] . Many positively charged lysines in histones are believed to have critical roles in this packaging process by neutralizing the negative change of phosphate in the DNA. However, the nucleosome structure occludes DNA from many cellular processes, including transcription, DNA replication and DNA repair. To enable dynamic access to the packaged DNA, cells have evolved a set of specialized chromatin remodelling complexes [2] . One class of remodelers including SWI/SNF, ISWI and CHD alters DNA packaging by sliding, ejecting, or reorganizing nucleosomes in an ATP-dependent manner. Another class achieves their function by adding or removing covalent modifications on histone tails. These post-translational modifications include methylation (me), acetylation (ac), monoubiquitylation (ub1) and so on [3] . Acetylation in particular negates the charge on ɛ-amino groups of lysine residues, therefore changing chromatin folding as the direct consequence of altering the histone–DNA or histone–histone electrostatic interactions. Some histone modifications exert their remodelling effects by recruiting chromatin remodelling factors. Importantly, acetylation can have both effects as it serves as a recognition site for the bromodomain, a motif common in ATP-dependent remodelers. It has been known for >40 years that there are multiple acetylation sites in the four core histones [4] . The levels of acetylation are regulated by two opposite enzymatic reactions that either transfers or removes the acetyl moiety of acetyl-CoA to the ɛ-amino group of lysine side chains. These reversible processes are performed by histone acetyltransferases (HATs) and histone deacetylases (HDACs) [5] . Acetylation has long been associated with transcriptional activation and HATs have been identified as transcriptional coactivators. In contrast, histone deacetylation is generally thought to have roles in transcriptional repression and HDACs have been identified as transcriptional corepressors [6] . Numerous in vitro acetylation assays and in vivo gene inactivation studies in past decades have suggested the existence of a specific regulatory mechanism based on the substrate specificity of HATs [7] . Based on these results, one would expect diverse genomic distribution patterns for different histone acetylation marks accompanied with preferential binding of each HAT or several HATs as the results of substrate specificity. On the contrary, the genome-wide mapping of 18 acetylation marks showed that they were targeted to enhancers, promoters and actively transcribed gene bodies with only subtle differences [8] . Also, the same approach demonstrated five HATs (p300, CBP, MOF, PCAF and Tip60) and four HDACs (HDAC1, 2, 3 and 6) were recruited to the hyperacetylated regions [9] , contradicting previous findings that HDACs are targeted primarily to transcriptionally inactive regions. In addition to the localization in active genes, HATs and HDACs were found to be transiently recruited to poised genes marked by H3K4 methylation for future activation [9] . Beyond studying their modifying enzymes or genomic locations, analysing the kinetics of these modifications has been proven to be very informative. We and others have measured the site-specific kinetics of histone methylation by quantitative mass spectrometry using stable isotope labelled methionine as a tracer [10] , [11] , [12] , [13] , [14] . As methionine can be metabolized to S -adenosyl methionine, the direct methyl group donor for the methylation reaction, the labelling is very efficient. By contrast, labelling acetylation is more difficult since cells use multiple metabolic pathways to generate acetyl-CoA. Dozens of studies in the past 30 years have used radioactive acetate as a tracer to estimate the turnover of acetylation on whole histones [15] , [16] , [17] . As summarized by Waterborg, these studies identified fast (half-life of few min.) and slow turnover rates (half-life of ~30 min.) in all four core histones from yeast to plant and animal cells [18] . However, these results provided an estimation of overall acetylation turnover in each core histone without site-specific information. In addition, these rates appear faster than would be needed to account for the rate observed for transcription [18] . To address these issues, we developed a new metabolic labelling method to study acetylation kinetics at specific lysines using quantitative target mass spectrometry via selective reaction monitoring (SRM) [14] . This first report of acetylation half-lives is selective for pools of old histone by virtue of a double labelling scheme and revealed a subset of sites that are surprisingly long-lived. Measurement of acetylation turnover in old histone Acetyl-CoA is generated from multiple sources, including glucose, pyruvate, glutamine and fatty acids. Using mammalian cells in culture, the main source of acetyl-CoA for histone acetylation was found to be citrate generated during glucose metabolism [19] . Therefore, we used 13 C 6 -glucose (simply referred to here as ‘heavy glucose’) as a source of isotope tracers that via acetyl-CoA would be introduced into the acetyl groups of histones [20] . However, the other sources of acetyl-CoA mean that only some fraction of the acetyl-CoA pool can be labelled by a single source, hence lowering the observed appearance rate of new acetyl groups. However, this effect can be mathematically modelled and the true appearance rate determined for reaching steady-state levels of labelled acetylation (Methods). We also investigated labelling using 2,3 13 C 2 -pyruvate (see below), but only achieved ~70% the labelling level of glucose which itself was near 80% ( Supplementary Fig. S1 ). Both reagents will be converted to acetyl-CoA with a +2 Da ‘label’ in acetyl groups that is transferred to lysine side chains ( Fig. 1b ). Our labelling scheme as shown in Fig. 1a includes two labelling steps. First, histones were exhaustively labelled by growing in media containing 13 C 6 —arginine for 7 days to label >90% histones so each of tryptic peptide produced from histones derivatized with propionic anhydride carries a +6 Da mass shift [14] . Second, cells were then switched to the media with regular arginine and heavy glucose (not supplemented with pyruvate or glutamine). After the media switch, all the acetylation being installed before the switch will have light acetyl group (referred as old ac) while the new acetylation will carry a +2 Da acetyl group (referred as new ac) in an ideal condition when acetyl-CoA is 100% labelled. Given the metabolic complexities of new histone synthesis on mixed isotopes, we limited our measurements to old histone that was synthesized before the media switch to track the rate of old acetyl groups being replaced by new ( Supplementary Methods ). 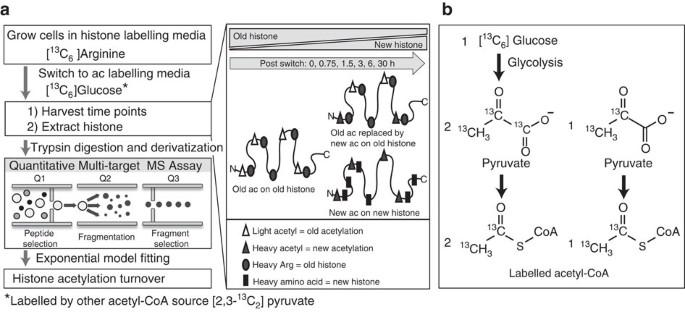Figure 1: Schematic of experimental workflow for the measurement of histone acetylation turnover. (a) The approach involves two steps of stable isotope labelling to detect old versus new acetylation events specifically on old histones. The workflow begins with exhaustive labelling of cells in heavy arginine media to label the histone backbone (depicted as a dark oval), followed by media exchange to label newly installed acetyl groups in lysine residues. Time points are taken and the material subjected to quantitative mass spectrometry (MS) analysis of histone peptides. Detection of old acetylation corresponding to a light acetyl group (depicted as a light triangle) and new acetylation with a heavy acetyl group (depicted as dark triangle) is followed by fitting the data to an exponential model to calculate acetylation turnover rate for each site. (b) Stable isotope labelled glucose (or sodium pyruvate) is converted to labelled acetyl-CoA by primary metabolism. Figure 1: Schematic of experimental workflow for the measurement of histone acetylation turnover. ( a ) The approach involves two steps of stable isotope labelling to detect old versus new acetylation events specifically on old histones. The workflow begins with exhaustive labelling of cells in heavy arginine media to label the histone backbone (depicted as a dark oval), followed by media exchange to label newly installed acetyl groups in lysine residues. Time points are taken and the material subjected to quantitative mass spectrometry (MS) analysis of histone peptides. Detection of old acetylation corresponding to a light acetyl group (depicted as a light triangle) and new acetylation with a heavy acetyl group (depicted as dark triangle) is followed by fitting the data to an exponential model to calculate acetylation turnover rate for each site. ( b ) Stable isotope labelled glucose (or sodium pyruvate) is converted to labelled acetyl-CoA by primary metabolism. Full size image Appearance of new acetyl in H3K14ac but not in H3K4ac Different from the ‘SILAC’ approach where stable isotopes are used to measure protein expression ratios [21] , we used them here to distinguish old versus new histone [22] while also initiating a temporal pulse of new acetyl-CoA in live cells ( Fig. 1a ). As shown in Fig. 2a , a fast appearance of new acetyl was observed in H3K14ac from old histone when the K9 in the same peptide was unmodified (H3K9un-K14ac). The +2 Da mass shift in new acetyl allows discrimination of new from old acetylation even in the 30 h sample with the least intense signals of all the six time points. This decrease in absolute intensity was due to dilution of old histone as the synthesis of new histone builds, consistent with previous observations [14] . Showing a striking difference at the other extreme, no new acetyl was observed for H3K4ac ( Fig. 2b ). The background level of noise for H3K4ac with new acetyl was steady over the entire 30 h time course. As histone peptides from similar cell numbers were subjected to quantitative multi-target mass spectrometry analysis, the fast increase of new acetylation accompanied by the fast decrease of old acetylation indicated a fast rate of turnover for H3K14ac. 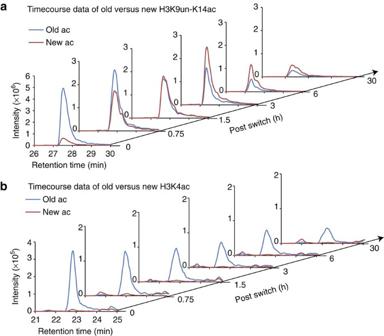Figure 2: Appearance of new acetylation on histone peptides detected by quantitative mass spectrometry. Shown on they-axes are the raw intensity values determined from the mass spectrometric data. The temporal profile for signals corresponding to old (blue) versus new (red) acetylation on the H3K9un-K14ac (a) and H3K4ac (b) peptides exhibiting fast and no turnover, respectively. Both old and new acetylation were quantified using total peak areas from three pairs of transitions (that is, precursor → fragment). Figure 2: Appearance of new acetylation on histone peptides detected by quantitative mass spectrometry. Shown on the y -axes are the raw intensity values determined from the mass spectrometric data. The temporal profile for signals corresponding to old (blue) versus new (red) acetylation on the H3K9un-K14ac ( a ) and H3K4ac ( b ) peptides exhibiting fast and no turnover, respectively. Both old and new acetylation were quantified using total peak areas from three pairs of transitions (that is, precursor → fragment). Full size image Fast increase of new acetyl in a subset of acetylation sites To account for slight variations in absolute loading amounts, two types of normalization schemes, called relative levels and distributive levels, were used in this paper (see formulas in the Methods section). Relative level is the signal for a new acetylation for a particular site normalized against the signals from all the modification states of the peptide that harbours that site (old histone only); distributive levels are simply the ratio of new versus (new+old) acetylation signals at a particular site. As shown in Fig. 3a , the relative levels of new acetylation determined for the 19 acetylation sites demonstrated two general types of behaviour. Ten of the sites showed robust increases in new acetylation: H3K9, H3K14, H3K18, H3K23, H3.1/2-K27, H3.3-K27, H2AK5, H2AK9, H4K5 and H4K16. The stable level of acetylation labelling at these sites ranged from 30–80% and was reached within 6 h for all ten sites. By contrast, no appearance of new acetylation was observed for the other nine acetylation sites ( Fig. 3a ; distributive levels are shown in Fig. 3b for all sites measured). 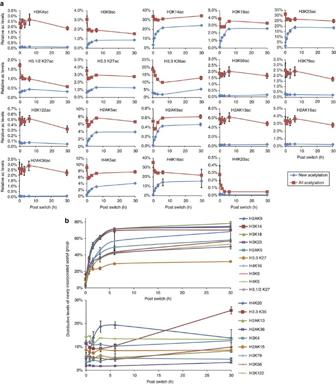Figure 3: Appearance of new acetyl group in 19 acetylated lysines using13C6-glucose as a tracer. (a) Relative levels of both new acetylation (occurred after the media switch; blue diamonds) and all acetylation (both old and new; red squares) in 19 acetylated sites. These levels were determined by normalizing against overall signal from all measured modfied species (see Methods). (b) Distributive levels of new acetylation for 19 acetylated sites were determined by divding the peak area of new acetylation by that of total acetylation present at each particular site. The ten fast sites reaching a steady plateau are shown in upper panel, while the sites with no detectable new acetylation are displayed in the lower panel. Data from two biological replicates with three technical replicates of each were reported with s.e.m. values shown as error bars. Figure 3: Appearance of new acetyl group in 19 acetylated lysines using 13 C 6 -glucose as a tracer. ( a ) Relative levels of both new acetylation (occurred after the media switch; blue diamonds) and all acetylation (both old and new; red squares) in 19 acetylated sites. These levels were determined by normalizing against overall signal from all measured modfied species (see Methods). ( b ) Distributive levels of new acetylation for 19 acetylated sites were determined by divding the peak area of new acetylation by that of total acetylation present at each particular site. The ten fast sites reaching a steady plateau are shown in upper panel, while the sites with no detectable new acetylation are displayed in the lower panel. Data from two biological replicates with three technical replicates of each were reported with s.e.m. values shown as error bars. Full size image System response and background levels The relative levels of all 19 sites showed a slight dip in the second time point (that is, t =45 min.) after the switch to new media at time zero. ( Fig. 3a ). Some sites reached stable levels immediately after the 90 min. point (such as H3K9 and H3K23), while other sites rose back more gradually to their stable levels (such as H3K18 and H2AK5). This slight dip in relative acetylation levels seems related to the experimental procedure of media change and buffer washing necessary for removal of heavy arginine and regular glucose present in the old media; an exact explanation will require further investigation. It is also worth noting that initial new acetylation levels are theoretically zero. Therefore, the observed presence of signal for new acetylation in several sites (for example, H3.1/2-K27ac, H3.3-K27ac, H3.3-K36ac, H3K79ac and H3K122ac) represent a baseline signal from unknown sources at ~10%; background levels for the other sites were <5% ( Fig. 3b ). Site-specific half-life of histone acetylation turnover As shown in Fig. 3b , three different kinetic patterns were found in the graphs of distributive levels and were therefore used to categorize acetylation sites. Group I, the 10 sites with fast increases of new acetylation levels (relative and distributive), had half-lives ranging from 0.8–2.3 h ( Table 1 ; also see Methods and Supplementary Fig. S2 for details of data fitting). It is worth noting that labelled population is only equal to the labelling efficiency of acetyl-CoA pool when all the population of this site is turned over. The fact that the labelled population varied among sites suggests the likely existence of the subpopulation with very low or no turnover in those sites having low levels of labelled population (such as H3K27ac). Table 1 Site-specific acetylation turnover and half-lives for 19 acetylation sites in core histones. Full size table The acetylation sites H4K20 and H3.3-K36 exhibited a distinct behaviour and were therefore classified separately as Group II ( Fig. 3 ). At these sites, there is a sharp reduction in the overall acetylation level, yet no appreciable new acetylation detected (see Fig. 3 panels for H4K20 and H3.3-K36). Also at these sites, increasing methylation contributed in part to the observed decrease of overall acetylation signal ( Supplementary Methods ). For Group III containing seven sites ( Table 1 ), no change of distributive levels of new acetylation was observed (that is, no evidence for acetylation turnover in the 30 h experiment; see Fig. 3b ). To further confirm our findings, we performed the same experiment using heavy pyruvate as the tracer. Despite dropping a few sites in the assay due to a lower labelling efficiency (~60% versus 80% for glucose) and higher noise levels, the overall trend is similar ( Supplementary Fig. S1 ). It is worth noting that all the peptides from histone H3 except H3K27-K36 were conserved among the three H3 variants (H3.1, H3.2, and H3.3); therefore results reported here represent the average turnover for these three variants. The levels determined are shown in Table 1 and ranked according to their turnover rate within Group I. Butyrate-induced acetylation is restricted to Group I sites To confirm our findings, we measured histone acetylation levels for all 19 sites in response to broad-spectrum HDAC inhibition. Both relative levels and fold changes were reported and the results shown in Supplementary Fig. S3 for the time course data obtained from cells treated with sodium butyrate. To avoid secondary effects from cell cycle arrest caused by butyrate treatment, the fold change of acetylation levels in 6 h of treatment was used in Table 1 for comparison to rates of turnover. Strikingly, only Group I sites showed between 2 and 10-fold increases in acetylation stoichiometry. In addition, the response to butyrate treatment showed a similar trend to the half-lives of fast turnover sites ( Fig. 4a ). All the Group III sites with no turnover showed <1.1 fold or lower response to butyrate. This strongly corroborates our kinetic findings that turnover of these sites is in fact extremely low. 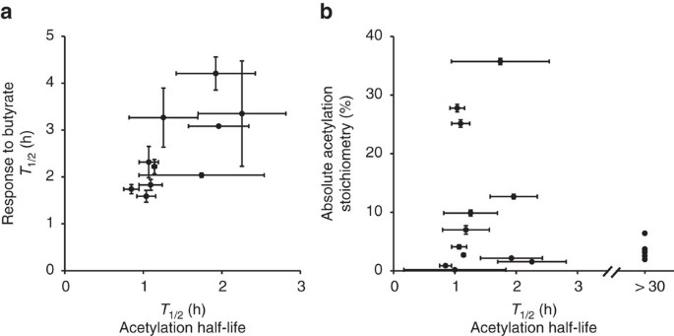Figure 4: Correlaton analyses of acetylation half-lives. (a) Half-lives of acetylation sites with fast turnover correlated with their response to treatment with sodium butyrate. (b) Correlation ofT1/2values with the absolute stoichiometry of acetylation for each site. Note that half-lives for sites with undetectable turnover were all set to >30 h (x-axis, lower right). Both vertical and horizontal error bars indicate the s.d. from their respective analyses. Figure 4: Correlaton analyses of acetylation half-lives. ( a ) Half-lives of acetylation sites with fast turnover correlated with their response to treatment with sodium butyrate. ( b ) Correlation of T 1/2 values with the absolute stoichiometry of acetylation for each site. Note that half-lives for sites with undetectable turnover were all set to >30 h ( x -axis, lower right). Both vertical and horizontal error bars indicate the s.d. from their respective analyses. Full size image An overall summary of the rates of acetylation turnover mapped onto sites on histone tails is provided in the Fig. 5 diagram. No correlation between turnover rate and the normal levels of acetylation was found except that the three most abundant acetylation sites (H3K14ac, 28%; H3K23ac, 25%; H4K16ac, 36%) all had fast turnover. Other than that, turnover rates for sites with low acetylation stoichiometry could be found in all three different groups ( Table 1 and Fig. 4b ). 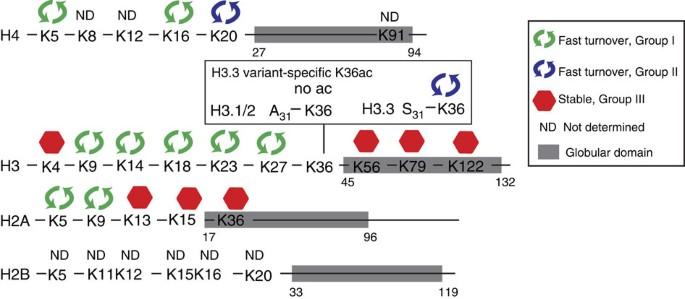Figure 5: Summary of acetylation turnover rates at 19 distinct lysine residues within core histones. Illustrations showing known lysine acetylation sites in four core histones as ‘K’ followed by amino acid residue number. The globular domains are marked by grey bars. Fast turnover sites are overlaid with green and blue arrows for Group I and II sites, respectively. Stable sites (Group III) are indicated by red stop signs. Sites not measured in this study are labelled as ND. Figure 5: Summary of acetylation turnover rates at 19 distinct lysine residues within core histones. Illustrations showing known lysine acetylation sites in four core histones as ‘K’ followed by amino acid residue number. The globular domains are marked by grey bars. Fast turnover sites are overlaid with green and blue arrows for Group I and II sites, respectively. Stable sites (Group III) are indicated by red stop signs. Sites not measured in this study are labelled as ND. Full size image Genome-wide mapping of HATs and HDACs by ChIP-seq have shown both of them are enriched in active genes and appear to positively correlate with transcription levels [9] . This suggests the removal of acetylation in active genes to reset chromatin modification after gene transcription. Such observations are consistent with a well-established model in Saccharomyces cerevisiae where the Rpd3S histone deacetylase complex is recruited to H3K36me2/3-decorated chromatin (methylated by Set2) to deacetylate nucleosomes behind elongating RNA Pol II to prevent cryptic initiation of transcription within the coding region [23] . In addition to deacetylation of nucleosomes within the gene body, the Set3 histone deacetylase complex can also be recruited by H3K4me2 (methylated by Set1) to deacetylate 5′ transcribed regions [24] . Different from yeast HDAC complex, the mammalian counterpart lacks the chromodomain for the direct targeting to H3K36me2/3 chromatin. However, both Tip60 and HDAC6 can be targeted to active genes through the interaction with Pol II (ref. 9 ). The likely outcome of targeting both HDACs and HATs to actively transcribed genes will be a high turnover rate of histone acetylation in these regions. Indeed, we observed very fast turnover in 12 acetylation sites (Group I and II, in Table 1 ) with half-lives ranging from 0.8 to 2.3 h. In addition, all these marks except H4K20ac have been shown to be localized in promoters/enhancers, and/or active transcribed gene bodies with positive correlations to transcriptional activity [8] . As mentioned in the Introduction, previous pulse/chase studies using radioactive acetate have determined overall acetylation of H3 and H4 to be as fast as 2–3 min. in the fast phase and ~30 min. in the slow phase. Considering the transcriptional elongation rate of 0.3–0.8 kb min −1 . determined in mammalian cells by imaging the transcription of a single gene [25] , it takes ~6–15 min to transcribe through a 5 kb small gene. With the additional time required for transcription initiation, it is improbable for one cycle of removal of acetylation in the gene bodies for all the genes to be as fast as several minutes. Therefore, it is possible that previous studies using radioactive acetate selectively labelled histones in highly transcribed genes during the short pulse due to a limited pool of labelled acetyl-CoA. This contrasts with our half-lives, determined with steady-state levels of acetyl-CoA as indicated by the stable population of labelled histones at each lysine in Group I. As shown in Fig. 3b , the highest labelling efficiency is ~80%, implying that at least 80% of acetyl-CoA pool is labelled by the glucose labelling scheme reported here. Seven sites showed no significant increase of new acetylation or decrease of old acetylation and were categorized as Group III as ‘no detectable turnover’. Except H3K4ac and H3K56ac, there are precious few functional studies to draw from for these Group III sites. Genome-wide mapping studies of H3K4ac in both human and S. cerevisiae have determined H3K4ac is localized at active gene promoters [8] , [26] . A genetic screen in yeast has determined deacetylation of H3K4 is mainly performed by Hst1 and Sir2 (to lesser extent) in euchromatin, and only dependent on Sir2 in heterochromatin [26] . Importantly, both Hst1 and Sir2 are NAD-dependent deacetylases belonging to the class III HDAC family. Acetylation within the globular core domain of histone H3 on K56 has been shown to have a critical role in packaging DNA into chromatin following DNA replication and repair in budding yeast [27] . Similar to H3K4ac, deacetylases of H3K56ac are also known to be NAD-dependent class III HDACs, namely Hst3 and Hst4 (refs 28 , 29 ). Very interestingly, a puzzling result has been reported recently that levels of H3K56ac were not affected by all the tested HDAC inhibitor targeting class I/II or class III (ref. 30 ). This result can be explained by our observation of extremely slow turnover of H3K56ac. In addition to Group III sites, some Group I sites might also have stable subpopulations. For example, H3K27ac from both canonical H3.1/2 and the H3.3 variant showed low labelling levels (30 and 20%, respectively), suggesting more than half of K27ac could be stable. The observation that acetylation turnover could be twofold faster when adjacent sites are both acetylated (that is, for K9/K14 on H3) but ~50% slower when the neighbouring site was methylated ( Supplementary Fig. S4 ) highlights the regulatory effects of nearby modifications. Such observations can be explained by either promiscuous behaviour of HATs and HDACs, or intentional recruitment or occlusion of such enzymes at specific genomic locations. The higher turnover of dual-acetylated H3 at both K9 and K14 could be caused by higher local HAT/HDAC concentrations in the chromatin region where they are present. In addition, the observation of H3.3 variant-specific K36ac suggested that its cognate HAT/HDAC pair(s) have superior substrate specificity capable of discriminating the single amino acid changed among the H3 variants in this region of sequence (localized five residues away from K36; see Fig. 5 , Supplementary Fig. S5a and Supplementary Methods ). With more genetic alterations of HATs being identified in cancers and the use acetylation modulators (for example, HDACi, HAT inhibitors, bromodomain inhibitors) increasing in cancer research [31] , the results described here provide a new context to understand and measure the pharmacokinetic behaviour of different acetylation sites in vivo . The importance of acetylation is not limited to histones, as it appears as widespread as phosphorylation in intracellular signalling [32] . It should not escape our attention that high efficiency metabolic labelling of acetyl-CoA provides a useful tool for functional studies of protein acetylation generally. For example, what is the turnover rate of acetylation in p53 when DNA damage is induced? Stable isotope tracer labelling and sample preparation HeLa S3 cells were grown in adherent for 7 days at 37 °C in heavy DMEM media (omission of arginine, AthenaES) supplemented with [ 13 C 6 ]arginine (99% enriched, Cambridge Isotope Laboratories) and 10% dialyzed fetal bovine serum before release into glucose and sodium pyruvate free DMEM plus 10% dialyzed fetal bovine serum supplemented with [ 13 C 6 ]glucose (2 gl −1 , 99% enriched, Cambridge Isotope Laboratories) or [2,3- 13 C 2 ] pyruvate (10 mM, 99% enriched, Cambridge Isotope Laboratories). Cells were washed twice with phosphate buffered saline to remove old media before releasing cells into new media. Stable isotope labelled cells were harvested at time points of 0, 0.75, 1.5, 3, 6 and 30 h after the media switch and 5 mM sodium butyrate treated cells at 0, 1.5, 3, 6 and 24 h before collection and flash freezing in liquid N 2 . Histones from acid extraction of isolated nuclei were derivatized using propionic anhydride and digested with trypsin, as described previously [14] , [33] . Nano-capillary liquid chromatography triple quadrupole mass spectrometry (nLC-QqQ MS) The digested and derivatized histone peptides were diluted in 0.1% TFA and injected to nLC-QqQ MS (Dionex nanoLC and a ThermoFisher Scientific TSQ Quantum). Peptides were first loaded to a trapping column (2 cm × 150 μm) and then separated with an analytical capillary column (10 cm × 75 μm). Both were packed with Magic C18 resin (Michrom). The chromatograph gradient was achieved by increasing percentage of buffer B from 2–35% at a flow rate of 0.35 μl min −1 (A: 0.1% formic acid in water, B: 0.1% formic acid in acetonitrile) over 40 min. The peptides were then introduced into QqQ MS by electrospray from an emitter with 10 μm tip (New Objective) as they were eluted from capillary column. The QqQ settings were as follows: collision gas pressure of 1.5 mTorr; Q1 peak width of 0.7 (FWHM); cycle time of 3.5 s; skimmer offset of 10 V; electrospray voltage of 2.6 kV. SRM method development and mass spectral data analysis SRMs capable of discriminating 19 acetylation sites from 13 different histone peptides were developed with two to four fragment ions for each species. Various histone peptides with different modifications were purchased or custom synthesized from Anaspec or Genescript to assist the method development. Data were analysed in Skyline with Savitzky–Golay smoothing [34] . All labelled and unlabelled peaks were grouped as a whole for manual peak determination to avoid bias. Total peak areas from SRMs were used for quantification (as listed in Supplementary Table S1 ). Peptide nomenclature and data handling All the peptides with their modifications that were quantified in this study are listed in Supplementary Table S1 . In this paper, we simply used the position of lysine that can be acetylated in the protein to refer the peptide. For example, T 3 KQTAR 8 was referred to as the ‘H3K4 peptide’ and K 9 STGGKAPR 17 as the ‘H3K9-K14 peptide’. For the purpose of determining acetylation turnover, three forms were measured for the peptide targeted by mono-acetylation (H3K56, H3K122 and H2AK36): unmodified (chemical derivatized by propionylation, +56 Da) and acetylated (light and heavy, +42 and +44 Da); six forms were measured for the peptide targeted by both acetylation (ac) and methylation (me) to the single lysine: unmodified, acetylated (light and heavy), me1, me2 and me3 (H3K4, H3K79 and H4K20); nine forms were measured for the peptide targeted by di-acetylation to two lysines (H3K18-K23, H2AK5-K9 and H2AK13-K15); 18 forms were measured for H3K9-K14 (K9 is methylated and acetylated, K14 is acetylated). Multiple channels of measurement were aggregated together for each site for those peptides with many modification states. For example, five channels of K14ac, with K9 carrying un, me1, me2, me3 or ac, were summed together to represent the total level of K14ac. Finally, for histone H4 we only measured H4K5ac and H4K16ac because the two internal acetylation sites (H4K8ac and H4K12ac) were difficult to measure with SRM. Two quantification schemes were used in this study, differed simply by which pool of peptides was used to normalize the signal for any given acetyl mark [10] , [14] . Distributive level is the term used to refer to the normalization of heavy acetylation within acetylation of each site (that is, the signal of heavy ac is divided by the combined signal of heavy plus light ac). Relative level is used to indicate signals from all the modification species found at a particular site are summed as total (ac site: unmodified+light ac+heavy ac; ac+me site: unmodified+me1+me2 +me3+light ac+heavy ac). Recall that heavy acetylation is new and light acetylation is old. Determination of acetylation turnover rates and half-lives An exponential decay model with three parameters was used to fit the data in Group I using the distributive levels of new acetylation (with all six time points). In the equation, new acetyl= P * (1-exp(- k * t ))+ n , p represents the labelled pool of acetylation in each site, k for the turnover rate, and n for the noise (initial value is not zero; see Supplementary Fig. S2a ). The curve fitting was implemented by the cftool software package in Matlab (version 7.10). A different model (total acetylation=a* exp(−k*t)+c) was used to fit the data in Group II using relative levels of total acetylation, where parameter a is for initial level of acetylation in old histone, c for stable level of acetylation and k for the turnover rate of deacetylation ( Supplementary Fig. S2b ). The half-life of turnover is calculated by ln2/k. How to cite this article: Zheng, Y. et al. Measurement of acetylation turnover at distinct lysines in human histones identifies long-lived acetylation sites. Nat. Commun. 4:2203 doi: 10.1038/ncomms3203 (2013).